Multimode quantum interference of photons in multiport integrated devices Photonics is a leading approach in realizing future quantum technologies and recently, optical waveguide circuits on silicon chips have demonstrated high levels of miniaturization and performance. Multimode interference (MMI) devices promise a straightforward implementation of compact and robust multiport circuits. Here, we show quantum interference in a 2×2 MMI coupler with visibility of V =95.6±0.9%. We further demonstrate the operation of a 4×4 port MMI device with photon pairs, which exhibits complex quantum interference behaviour. We have developed a new technique to fully characterize such multiport devices, which removes the need for phase-sensitive measurements and may find applications for a wide range of photonic devices. Our results show that MMI devices can operate in the quantum regime with high fidelity and promise substantial simplification and concatenation of photonic quantum circuits. Quantum technologies aim to harness superposition and entanglement to enhance communication security [1] , provide exponential computational advantage for particular tasks [2] , [3] , including factoring [4] , database search [5] and simulation of important quantum systems [6] , and reach the ultimate limits of precision in measurement [7] . Photons are an appealing information carrier for their inherently low-noise, high-speed transmission, and the fact that entangling interactions between photons can be achieved using only linear optical circuits [1] , [8] , [9] , [10] or mediated by atom-like systems [12] , [13] . A photonics approach to these technologies requires complex, multiport quantum circuits—essentially multipath, multiphoton interferometers—that exhibit high fidelity quantum interference. Circuits fabricated from 2×2 directional couplers have demonstrated high performance [13] , [14] , [15] , [16] , [17] ; however, construction of more sophisticated multiport circuits would require their decomposition into a very large number of 2×2 directional couplers. For example, an arbitrary N × N mode unitary [18] would require a sequence of O ( n 2 ) individual 2×2 directional couplers. Multimode interference (MMI) devices are based on the self-imaging principle, by which an input field profile is reproduced in single or multiple images at periodic intervals along the propagation direction of a multimode waveguide [19] , [20] . The effect is based on the propagation properties of a guide with a large number of lateral modes that see different effective refractive indices. Each mode propagates at a specific velocity accumulating different phases that results in constructive and destructive interference along the multimode region. At the position in which all the modes re-phase the total electromagnetic field is the same as the input, resulting in a self-imaged condition. MMI devices allow the design of N × M splitters with superior performances, excellent tolerance to polarization and wavelength variations, and relaxed fabrication requirements compared with the other main beam-splitting technology, the directional couplers. Consequently, MMI couplers have found applications in a broad range of photonic systems [21] , including phase diversity networks, light switching and modulators, in laser architectures and for optical-sensing applications. In the context of photonic quantum circuits, they promise to dramatically reduce the complexity of such circuits, including for example those required to generate maximally entangled path or 'NOON' states [22] , W states [23] and the implementation of N×N unitaries [18] . In contrast to directional couplers, the self-imaging effect in MMIs allows the flexibility to directly realize symmetric N×N multiport devices with several input and output ports. Multiport circuits are particularly promising for quantum optics and information purposes, and fundamental experiments have been conducted to study the behaviour of non-classical interference of single photons in bulk optics [24] and fibre [25] circuits. However, their performance is limited by stability and control of the splitting ratios. The implementation of multiport splitters in MMI devices should allow higher performances because of the monolithic and scalable architecture. However, it is not clear that the multimode nature of MMI devices will allow quantum operations, in particular quantum interference. Quantum interference with two photons is a defining distinction between classical and quantum states of light and is the key phenomenon that drives photonic quantum technologies. Quantum interference occurs when different quantum mechanical outcomes are indistinguishable. In the case of two photons entering the two input ports of a symmetric 2×2 unitary beamsplitter (one photon per input port), the outcomes of 'both photons reflected' and 'both photons transmitted' are indistinguishable. In this case, the interference is destructive so that the photons never leave in the two separate outputs, but a superposition of two photons in each output. This behaviour is in stark contrast to the case of two classical particles that would have a probability of 1/2 to leave in separate outputs. When the relative arrival time of the two photons is scanned, a characteristic Hong Ou Mandel (HOM) dip is observed [26] , because the classical probability of 1/2 holds for finite delay and the quantum probability of zero holds for zero delay. The width of this HOM dip is given by the coherence time of the photons. The visibility V ∈ [0, 1] of the dip (how close it gets to zero) is a measure of the degree of quantum interference. Any information that distinguishes the two probability amplitudes—for example, the photons have different polarizations, frequency, bandwidth and so on—reduces V <1. In this paper, after a description of the devices fabrication and the experimental setup, we report our results on a 2×2 MMI. Then we show operation of a 4×4 MMI with single photon pairs injected in all possible pairs of input ports. Finally, we describe and apply a technique to characterize the 4×4 device based on the measured HOM dip visibilities. Device design and fabrication MMI devices, including 2×2 and 4×4 couplers, were designed and simulated using a commercial beam propagation package ( Fig. 1b ). They were fabricated on a 4′′ silicon wafer, onto which a 16 μm lower cladding layer of thermally grown undoped silica was deposited, followed by a 3.5 μm core layer of silica doped with germanium and boron oxides deposited by flame hydrolysis. This core layer was patterned into 3.5-μm-wide single mode and 15 and 29-μm-wide multimode waveguides via standard optical lithographic techniques and then overgrown with a 16 μm upper cladding of phosphorus and boron-doped silica, with a refractive index matched to that of the lower cladding; simulations indicated single mode operation at 780 nm. The devices are composed of N single mode waveguides that serve as input and output for the multimode section and terminate with a separation of 250 μm at the edges of the device to allow input and output coupling with a polarization-maintaining fibre array. The coupling losses between fibres and chip were estimated to be 0.79 dB per facet. The 2×2 MMIs are composed of two input and two output waveguides that have a separation of 11 μm at the interface of the single mode and multimode region. The multimode region measures 1,090×15 μm. In the case of the 4×4 MMIs, the waveguides are separated by 8 μm at the interface to the multimode section, which measures 1,770×29 μm. 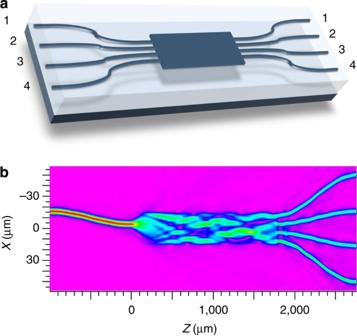Figure 1: MMI devices. (a) Schematic representation of a 4×4 MMI integrated chip. (b) Simulation of classical light propagation in the device shown schematically ina. Light is launched into input waveguide 2, and MMI in the central region results in equal intensity in each of the four output waveguides, via self imaging. Analogous behaviour is observed for injection of light in each of the other input waveguides. Figure 1: MMI devices. ( a ) Schematic representation of a 4×4 MMI integrated chip. ( b ) Simulation of classical light propagation in the device shown schematically in a . Light is launched into input waveguide 2, and MMI in the central region results in equal intensity in each of the four output waveguides, via self imaging. Analogous behaviour is observed for injection of light in each of the other input waveguides. 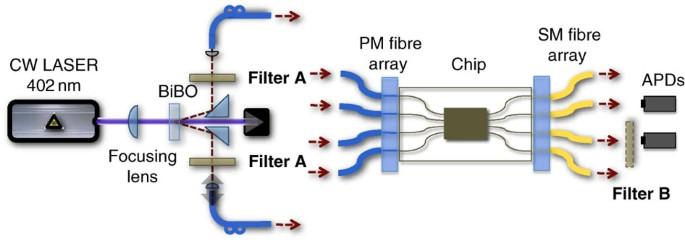Figure 2: Experimental setup for two photon quantum interference measurements in MMI devices. The parametric down-conversion source includes two Filter A (2nm FWHM in the 2×2 MMI measurements, 0.5nm FWHM in the 4x4 MMI measurements) to ensure single photons are indistinguishable. To increase the coherence length of the photons in the 2×2 MMI measurement, Filter B (0.5nm FWHM) was inserted the setup. CW, continuous wave; BiBO, bismuth borate; PM, polarization-maintaining; SM, single mode; APDs, silicon single-photon avalanche photodiodes. Full size image Experimental setup We measured quantum interference in MMI devices using single photon pairs produced in the spontaneous parametric down-conversion source shown schematically in Figure 2 . A type-I bismuth borate crystal pumped with a 60 mW continuous wave laser diode at 402 nm produced 804 nm pairs of photons. These photons were collected into single mode polarization-maintaining fibres after passing through 2 nm filters. The source was constructed in such a way that quantum interference with V ≈98.5% was routinely observed, confirmed with a directional coupler that has previously exhibited V =1 (ref. 16 ). Figure 2: Experimental setup for two photon quantum interference measurements in MMI devices. The parametric down-conversion source includes two Filter A (2nm FWHM in the 2×2 MMI measurements, 0.5nm FWHM in the 4x4 MMI measurements) to ensure single photons are indistinguishable. To increase the coherence length of the photons in the 2×2 MMI measurement, Filter B (0.5nm FWHM) was inserted the setup. CW, continuous wave; BiBO, bismuth borate; PM, polarization-maintaining; SM, single mode; APDs, silicon single-photon avalanche photodiodes. Full size image 2×2 MMI Any linear optical component can be described by a transition matrix M that maps input fields to output fields. Ideally, a balanced 2×2 MMI splitter should perform the same operation as a 2×2 directional coupler with a unitary matrix that describes the evolution from input to output [14] : which equally superposes the two modes. This is equivalent to the Hadamard operation with a phase shift (in the 2×2 case, there is only one equivalence class of symmetric splitters, this corresponds to the fact that different physical implementations can have different external phase relations, but the general description of the transformation is dictated by the unitary evolution [27] ). 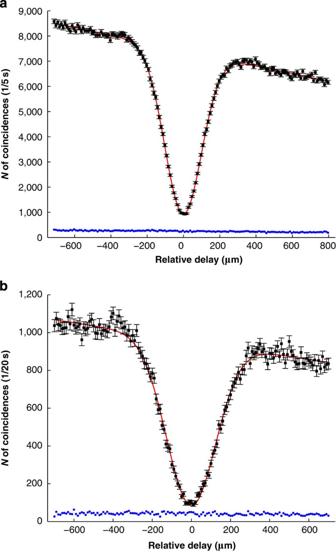Figure 3: Quantum interference in a 2×2 MMI coupler. (a) The measured HOM dip for 2 nm filters, corresponding to a dip FWHM of 239 μm. (b) The measured HOM dip for the same device and source, but with an additional 0.5 nm filter inserted into one output, resulting in a dip FWHM of 296 μm. Error bars are given by Poissonian statistics. The blue data show the measured rate of accidental counts. The visibilities for the 2×2 MMI, reported in the main text, are corrected for these accidentals. We observed the HOM dip shown in Figure 3a in a 2×2 MMI coupler. These data provide conclusive evidence that quantum interference does indeed occur in a MMI device (the linear slope in these data is due to decoupling of the input fibre as the timing delay is changed). However, the measured V =90.4±0.4% is significantly lower than the V ≈98.5% obtainable from the spontaneous parametric down-conversion source. The reason is that the propagation in the multimode section of the MMI introduces some distinguishability between the photons. We experimentally ruled out spatial, spectral and polarization mismatch of the photons, implicating the temporal degree of freedom. The different modes in the multimode section of the device have different effective refractive indices, which introduces a jitter in the time of flight of the photons from the input to the output waveguides, providing 'which path' distinguishing information, and thereby reduce V . Figure 3: Quantum interference in a 2×2 MMI coupler. ( a ) The measured HOM dip for 2 nm filters, corresponding to a dip FWHM of 239 μm. ( b ) The measured HOM dip for the same device and source, but with an additional 0.5 nm filter inserted into one output, resulting in a dip FWHM of 296 μm. Error bars are given by Poissonian statistics. The blue data show the measured rate of accidental counts. The visibilities for the 2×2 MMI, reported in the main text, are corrected for these accidentals. Full size image To confirm that this temporal jitter effect is the origin of the reduced visibility, we inserted a narrower 0.5 nm filter (as indicated in Fig. 2 ) in one of the output modes between the device and the detector, that is, not affecting the properties of the photon source, but simply increasing the coherence length of the photons. The additional filter acts as a quantum eraser [28] that erases the timing information by increasing the coherence time of the photons. Under these experimental conditions, we observed the HOM dip plotted in Figure 3b in the same 2×2 MMI device. In this case, V =95.6±0.9%, which confirms that timing jitter limits the visibility for the data shown in Figure 3b (the larger error bar is due to the lower count rate with the narrower filter). These data confirm that quantum interference occurs in MMI devices, and that the coherence length of the photons must be sufficiently long compared with the timing jitter that is introduced as a result of the different refractive indices of the MMI modes. While MMI devices are typically regarded as suitable devices for broadband operation—the reflectivity ratio is almost constant over a large wavelength range (±2% over a wavelength range of 50 nm)—our results show that the multimode propagation demands a narrow-band single photon wavepacket for quantum interference, but will operate identically with such narrow-band wavepackets across a broad wavelength range. 4×4 MMI Interestingly, the description of multiport splitters grows in complexity with N . For N ≤3, all symmetric N × N splitters can be described by one equivalence class, as the requirement on the conservation of energy defines the matrix to within external phases on the input and outputs. However, when N ≥4, there exists an infinite number of distinct equivalence classes [29] , and internal free phases are independent of the conservation of energy [22] . The transition matrix that describes an ideal symmetric 4×4 MMI splitter is: where θ is the free internal phase. In general, two different physical implementations would correspond to a different equivalence class and a different value of θ . In the case of a MMI splitter, the value of the internal phase is, in principle, dictated by the self-imaging condition [21] . However, the presence of fabrication imperfections in the device would drive the multimode section away from exact self-imaging, and the relation between the optical phases would deviate from the expected value. Moreover, the presence of unavoidable losses in the MMI coupler corresponds to the presence of additional optical modes in the transition matrix of the splitter, thus making the reduced 4×4 transition matrix M more complicated than equation (2). In principle, M could be reconstructed using a number of phase-sensitive measurements. Such measurements are, however, difficult in practice because of the need to maintain subwavelength stability in interferometers consisting of waveguide and fibre and/or free space paths. We have developed a technique to overcome this using only intensity measurements and two photon quantum measurements, but no phase-sensitive measurements, as described below. In contrast to the 2×2 MMI device in which quantum interference is destructive, in the 4×4 MMI device, interference between indistinguishable outcomes can be constructive for some of the 36 possible input and output combinations [24] . We characterized the quantum operation of a 4×4 MMI splitter by inputing the state |11〉 ij —a single photon in each input waveguide i and j . We considered all six combinations of two photons in four inputs, where i ≠ j (we did not consider the case of both photons in the same input as this does not give rise to quantum interference—such measurements provide no more information than bright intensity measurements do). As in the case of the HOM dip, quantum interference is revealed in the correlations in the output probability distribution. The probability to detect one photon in each output k and l , when two indistinguishable photons are injected into inputs i and j , is given by: where δ ij is Kronecker's delta and M ij is the element of the transition matrix. In the case of two distinguishable photons (equivalent to the classical analogue), the probability is given by and there is no interference between the two terms. Measurement of the generalized non-classical interference between two photons enables the reconstruction of the matrix M via measurement of the detection probabilities Q kl ij and C kl ij as described below. 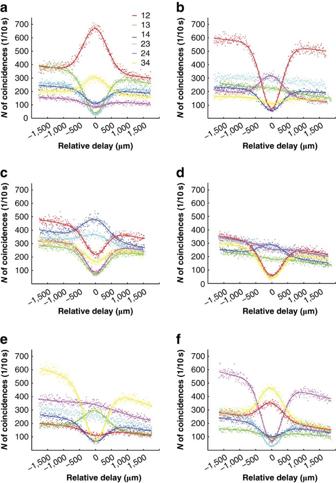Figure 4: Quantum interference in a 4×4 MMI coupler. Coincidence counts of two photons at the output ports of a 4×4 MMI device as the arrival time of the photons is varied. The different graphs represent the six possible input states in the splitter: (a) |11〉12, (b) |11〉13, (c) |11〉14, (d) |11〉23, (e) |11〉24, (f) |11〉34. The FWHM of∼800 μm is as expected for the 0.5 nm interference filters used. The visibilities for the 4×4 MMI, reported in the main text, are not corrected for accidentals. Figure 4 shows the rate of detecting two photons at the six possible output pairs of waveguides, for each of the six different input states of a 4×4 MMI splitter, as a function of the relative arrival time of the photons. For some input–output combinations, these data exhibit clear interference dips, analogous to the HOM dip. However, for other combinations, there are peaks and essentially straight curves. These behaviours are the result of the phase values of the matrix M and are conveniently summarized by plotting the visibility of the non-classical peak or dip, given by: where positive values indicate a dip and negative values a peak. 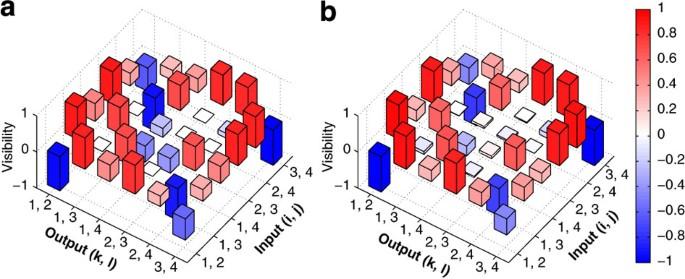Figure 5: Quantum interference matrix of a 4×4 MMI coupler. Measured (a) and reconstructed (b) visibility matricesVijklof the non-classical interference between two photons injected in input waveguidesiandjand detected in output waveguideskandlof a 4×4 MMI splitter. Positive visibilities correspond to a HOM-like dip, negative to peaks. The errors of the measured visibilities vary between 1.3 and 3.6%. Figure 5a shows the 6×6 matrix of measured visibilities V m obtained from the data of Figure 4 . Figure 4: Quantum interference in a 4×4 MMI coupler. Coincidence counts of two photons at the output ports of a 4×4 MMI device as the arrival time of the photons is varied. The different graphs represent the six possible input states in the splitter: ( a ) |11〉 12 , ( b ) |11〉 13 , ( c ) |11〉 14 , ( d ) |11〉 23 , ( e ) |11〉 24 , ( f ) |11〉 34 . The FWHM of ∼ 800 μm is as expected for the 0.5 nm interference filters used. The visibilities for the 4×4 MMI, reported in the main text, are not corrected for accidentals. Full size image Figure 5: Quantum interference matrix of a 4×4 MMI coupler. Measured ( a ) and reconstructed ( b ) visibility matrices V ijkl of the non-classical interference between two photons injected in input waveguides i and j and detected in output waveguides k and l of a 4×4 MMI splitter. Positive visibilities correspond to a HOM-like dip, negative to peaks. The errors of the measured visibilities vary between 1.3 and 3.6%. Full size image Reconstruction of the transition matrix We have developed a technique that uses only the values V ijkl and the classical intensity ratios | M ik | 2 to reconstruct the (reduced) transition matrix that describes the MMI device, assuming linearity of the device. To do this, we numerically search for a matrix M r that minimizes the root mean square distance between the experimentally measured V m and the reconstructed V r that corresponds to M r (see Methods section). The classical intensity ratios | M ik | 2 were measured using a multimode fibre at the output of the integrated chip and normalized to the power transmitted through a straight waveguide (that is, with no device). The uncertainty on this measurement, mainly given by input/output coupling, was estimated to be 2%. The numerical optimization produces The quality of the reconstructed transition matrix M r is confirmed by comparing the measured V m and calculated V r matrices in Figure 5 . From the measured values of classical intensity transmissions, it is clear that this MMI device does not operate as a 4×4 symmetric splitter. This moves the phase θ and shape of the matrix in equation (2) away from the value dictated by self-imaging condition. As the matrix of the visibilities is not normalized, we cannot benchmark the reconstruction using a standard definition of fidelity. We measured the quality of the reconstruction with a similarity [30] , [31] defined as S =1−∑| V r − V m |/2 n , where n =36 is the number of matrix elements. S can range from 0 (completely anti-correlated) through 0.5 (completely uncorrelated) to 1 (perfect overlap). We obtained S =95.6%. Additional optimization routines were performed with different initialization parameters to confirm that the measured transmissivities do indeed provide a good starting condition for the matrix M r . Our method to reconstruct the transition matrix can be used for any unknown linear optical element even in the case of losses. It is possible to calculate the reduced n × m transition matrix even in the case of large N × N ( N > n , m ) networks in which only n input and m output modes are accessible for measurements. Interestingly, the computation of the photon distribution at the output of a multiport circuit with many photons is a hard problem to solve from a computational perspective. The coincidence probability distribution is related to the permanent of the matrix that describes the multiport device [32] . As the calculation of the permanent of a matrix is a computationally difficult problem, the measurement of the coincidence probabilities in a device with many photons and many ports could represent a feasible implementation of quantum simulation that uses the bosonic nature of the photons to realize a hard computation. In general, it is possible to map the calculation of the permanent to the detection of multiphoton coincidences in the appropriate splitter. Although the form of the transition matrix that characterizes the MMI device is in principle fixed by the self-imaging condition, and no reconfigurability is possible, the data presented here on a 4×4 MMI splitter are the first small-scale example of such a quantum computation [33] . Multiphoton inputs to multiport devices are not only an essential ingredient of future photonic quantum technologies, but also enable the study of a rich variety of quantum interference phenomena [34] . The increasing need for more complex photonic networks will present the problem of the characterization of such integrated circuits and their imperfections. As demonstrated here, it is possible to take advantage of the properties of quantum states of light to reconstruct the behaviour of a photonic network, without the need for complex phase stable measurements. In the case of quantum networks, MMI devices promise to dramatically simplify and miniaturize the implementation of quantum circuits because of the possibility of performing complex multimode evolution of many photons in a single compact device. Reconstruction of the transition matrix The optimal transition matrix, defined as the matrix that minimizes the quantity , was reconstructed in two steps. We first fixed the classical intensity ratios and let the phases change; in the second step, both classical ratios and phases were optimized. To determine the standard deviation of the elements of M r , we repeated 5,000 iterations. The standard deviation for the absolute value of the matrix elements are: How to cite this article : Peruzzo, A. et al . Multimode quantum interference of photons in multiport integrated devices. Nat. Commun. 2:224 doi: 10.1038/ncomms1228 (2011).